Two-dimensional superconductivity at a Mott insulator/band insulator interface LaTiO3/SrTiO3 Transition metal oxides show a great variety of quantum electronic behaviours where correlations often have an important role. The achievement of high-quality epitaxial interfaces involving such materials gives a unique opportunity to engineer artificial structures where new electronic orders take place. One of the most striking result in this area is the recent observation of a two-dimensional electron gas at the interface between a strongly correlated Mott insulator LaTiO 3 and a band insulator SrTiO 3 . The mechanism responsible for such a behaviour is still under debate. In particular, the influence of the nature of the insulator has to be clarified. In this article, we show that despite the expected electronic correlations, LaTiO 3 /SrTiO 3 heterostructures undergo a superconducting transition at a critical temperature T c onset ~300 mK. We have found that the superconducting electron gas is confined over a typical thickness of 12 nm and is located mostly on the SrTiO 3 substrate. Perovskites-based structures including transition metal oxides have attracted much attention in the past decades, with the discovery of high- T c superconductivity and colossal magnetoresistance [1] . More generally, these compounds exhibit various electronic orders, going from the canonical anti-ferromagnetic (AF) Mott insulator when the onsite repulsion is maximum because of strong electronic interactions, to Fermi liquid-like metals when carrier doping is such that screening prevents the system from localization. Depending on the cations and the doping level involved, charge, spin and orbital orders can appear in the ground state together with metallic and even superconducting phases. Transitions between these states can be tuned by temperature, magnetic or electric fields [2] . All these compounds can be seen as stacks of oxide layers where the charge neutrality is conserved in the unit cell (u.c. ), but not necessarily in each layer. Therefore, the translation symmetry is locally broken at the interface and charge imbalance can develop. Like in band-gap engineering with semiconductors, it is possible to create artificial interface materials by growing thin layers of a transition metal oxide on top of another one. Recently, the observation of two-dimensional (2D) superconductivity [3] and magnetic correlations [4] at the interface between the two band insulators LaAlO 3 and SrTiO 3 has drawn a lot of attention. Another particularly interesting candidate is the homo-metallic structure LaTiO 3 /SrTiO 3 that uses TiO 2 plans as a building block [5] , [6] . Titanium is in the 3 d 0 state in the SrTiO 3 layer which is a band insulator of 3.2 eV bandgap, whereas it is 3 d 1 in the LaTiO 3 one which is therefore an AF Mott insulator due to strong correlations [7] . Providing the interface layer is TiO 2 , an extra electron is left in the structure every 2 u.c. [8] , [9] . As shown by photoemission [10] and optical studies [11] , a two-dimensionnal electron gas (2-DEG) develops and extends a few u.c. beyond the interface. Several theoretical approaches pointed out that an electronic reconstruction leads to an increase of the electronic density at the LaTiO 3 /SrTiO 3 interface [8] , [9] , [12] , [13] . Okamoto and Millis [8] proposed a phase diagram where different orbital and magnetic states occur as a function of the thickness of the LaTiO 3 layer and the strength of the Mott-Hubbard parameter U/t ( U is the Coulomb onsite repulsion energy, and t the hopping term between neighbour Ti sites). Fully polarized ferromagnetic metallic sub-bands are expected to form for thickness below 5 u.c. and U/t~ 8–10. However, Kancharla and Dagotto, [14] taking into account both local and long-range Coulomb interactions, showed that strong AF fluctuations reminiscent of the magnetic order of the bulk compound persist in the metallic phase. As suggested by Larson [15] and Okamoto [16] , lattice relaxation at the interface strongly modifies the band configuration, and may enhance the electronic correlations in the 2-DEG [12] . In this context, it is clear that the LaTiO 3 /SrTiO 3 interface layer appears to be a unique system to study the physics of a 2-DEG influenced by strong electronic correlations. In this study, we show that this heterostructure undergoes a superconducting transition and we are able to characterize the 2-DEG as extending mostly towards the SrTiO 3 side of the interface. Low-temperature transport measurements We have grown epitaxial layers of LaTiO 3 using pulsed laser deposition (PLD) on single crystal substrates of SrTiO 3 cut along (100) and (110) crystallographic directions. The details of the growth conditions and X-ray characterizations are given in Methods section and in Supplementary Figures S1 and S2 . In this study, we focus mainly on two LaTiO 3 /(100)SrTiO 3 heterostructures whose thickness of 40 and 60 Å correspond to 10 and 15 u.c. respectively. The sheet resistance measured in a Van der Pauw geometry decreases with temperature, indicating a metallic behaviour of the interface ( Fig. 1 ). At temperatures lower than 20 K the two samples exhibit an increase of resistance characteristic of weak localization in disordered 2D films. The heterostructures undergo a superconducting transition at T c onset ≈310 mK for the 10 u.c. sample and at T c onset ≈260 mK for the 15 u.c. sample (inset, Fig. 1 ). Thinner 5 u.c. (100) films and 20 to 100 u.c. thicker (100) films as well as (110) oriented films are not metallic at low temperature. 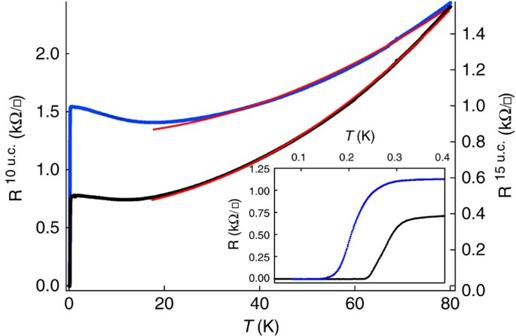Figure 1: Sheet resistance of the hererostructures. Sheet resistance a of the 10 u.c. (black dots, left axis) and 15 u.c. (blue dots, right axis) LaTiO3/SrTiO3samples in an intermediate range of temperature.The red lines correspond to quadratic fits of the formR(T)=AT2+R0. (Inset) Sheet resistance as a function of temperature showing the superconducting transitions atTconset=310 mK for the 10 u.c. (black dots) andTconset=260 mK for the 15 u.c. (blue dots), whereTconsetis defined by a 10% drop of the resistance. Figure 1: Sheet resistance of the hererostructures. Sheet resistance a of the 10 u.c. (black dots, left axis) and 15 u.c. (blue dots, right axis) LaTiO 3 /SrTiO 3 samples in an intermediate range of temperature.The red lines correspond to quadratic fits of the form R ( T )= AT 2 + R 0 . (Inset) Sheet resistance as a function of temperature showing the superconducting transitions at T c onset =310 mK for the 10 u.c. (black dots) and T c onset =260 mK for the 15 u.c. (blue dots), where T c onset is defined by a 10% drop of the resistance. 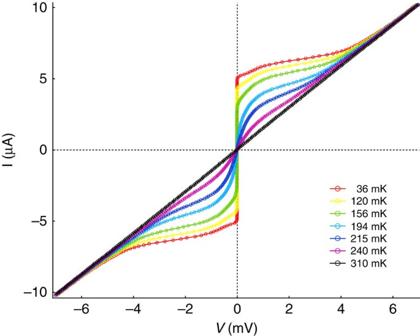Figure 2: Current–voltage characteristics of the 10 u.c. sample. The critical current at low temperature is 5 μA corresponding to a critical current per unit width of 16.7 μA cm−1. Full size image In Figure 2 , we show the current–voltage characteristics of the 10 u.c. sample measured at different temperatures. At low temperature, the I (V) curves show a clear critical current I c of 5 μA corresponding to a critical current per unit width of 16.7 μA cm −1 . For current much higher than I c , the I (V) curves merge together on a linear Ohmic law with a resistance corresponding to the normal resistance. In the case of the 15 u.c. sample, the critical current per unit width is found to be 14 μA cm −1 . 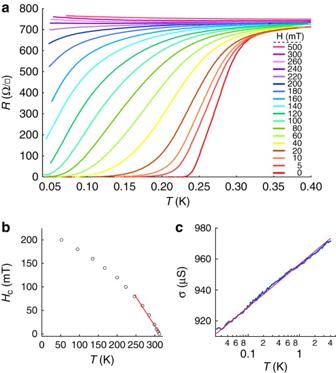Figure 3: Sheet resistance of the hererostructures under magnetic field. (a) Sheet resistance of the 10 u.c. sample as a function of temperature for different values of the perpendicular magnetic field. (b) Temperature dependence of the perpendicular critical field, defined as the magnetic field that suppresses 90% of the resistance drop. The red line indicates the linear dependence of the critical field with temperature close toTc. (c) Conductivity of the 15 u.c. sample as a function of temperature for a perpendicular magnetic field corresponding to the critical field. The red line corresponds to the expressionwithp=0.97 indicating that phase coherence is limited by electron–electron scattering (p=1)19. Figure 3a shows the sheet resistance of the 10 u.c sample as a function of temperature measured for different values of a magnetic field applied perpendicularly to the sample. The magnetic field induces a transition from a superconducting state to a nonsuperconducting one. The dependence of the critical field as a function of temperature is linear close to T c , which is consistent with the form taking into account a Landau–Ginsburg in-plane coherence length ( Fig. 3b ). The critical field extrapolated at T =0 is mT for the 10 u.c. sample and mT for the 15 u.c. sample (see Supplementary Fig. S3 ). At T =0, we found and . Measurements performed in a parallel magnetic field geometry give for the 10 u.c sample and for the 15 u.c sample. We thus extract the thickness of the 2D superconducting electron gas d 15u.c. =12 nm and d 15u.c. =13.5 nm. Note that this is an upper bound given the precision of the sample alignment in the parallel magnetic field. These values are close to the ones reported in LaAlO 3 /SrTiO 3 heterostructures [17] , [18] . In disordered electronic system, weak localization produces a decrease of conductivity that can be experimentally revealed by varying the temperature. In the particular case of a 2D system, the conductivity takes the remarkable logarithmic dependence with temperature , where p depends on the process that limits the phase coherence; p =3 for electron–phonon scattering and p =1 for electron–electron scattering in the dirty limit [19] . Such logarithmic temperature dependence is observed on our samples (see Fig. 3c ), thus confirming the 2D nature of the electron gas. The fit gives p =0.97±0.05 showing that the phase coherence is limited mainly by electron–electron scattering. Figure 2: Current–voltage characteristics of the 10 u.c. sample. The critical current at low temperature is 5 μA corresponding to a critical current per unit width of 16.7 μA cm −1 . Full size image Figure 3: Sheet resistance of the hererostructures under magnetic field. ( a ) Sheet resistance of the 10 u.c. sample as a function of temperature for different values of the perpendicular magnetic field. ( b ) Temperature dependence of the perpendicular critical field, defined as the magnetic field that suppresses 90% of the resistance drop. The red line indicates the linear dependence of the critical field with temperature close to T c . ( c ) Conductivity of the 15 u.c. sample as a function of temperature for a perpendicular magnetic field corresponding to the critical field. The red line corresponds to the expression with p =0.97 indicating that phase coherence is limited by electron–electron scattering ( p =1) [19] . Full size image Hall effect measurements. To investigate the density and mobility of charge carriers, we performed Hall measurements at low temperature ( Fig. 4 ). The experiment confirms that the sign of the hall coefficient is negative for both samples, indicating that electron-like charge carriers dominate the transport. The sheet carrier density was found to be 2 × 10 14 cm 2 for the 10 u.c. sample and 2.7 × 10 13 cm 2 for the 15 u.c. one. Taking the sheet resistance measured previously, we obtained a Hall mobility of 52 cm 2 V −1 s −1 for the 10 u.c. sample and 210 cm 2 V −1 s −1 for the 15 u.c. one. In an ideal picture, the interface between SrTiO 3 and LaTiO 3 can be observed as a Ti ions network, in the 4 + state in SrTiO 3 and in the 3 + one in LaTiO 3 . Therefore, one electron is left every two cells on average at the interface, which corresponds to an areal density of approximately 3 × 10 14 cm −2 (refs 8 , 9 ). This is approximatively the electron density measured through Hall effect in the 10 u.c. sample (2 × 10 14 cm −2 ), consistent with the value observed in LaTiO 3 /SrTiO 3 superlattices [6] by measuring the number of Ti 3+ in the vicinity of the interface. Optical studies confirm that free carriers with densities of approximately 3 × 10 14 cm -2 do exist in similar superlattices, with a typical mobility of 35 cm 2 /V −1 s −1 and an effective mass m * ≃ 2 m e [11] . The mobility that we measured on the 10 u.c. sample (52 ) is close to this value, which supports an effective mass close to 2 m e . The 15 u.c. has a lower sheet density of 2.7 × 10 13 cm -2 and a T c onset of only 260 mK. 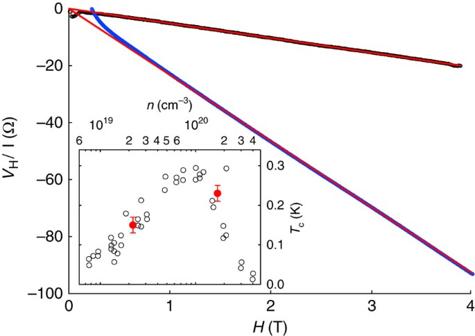Figure 4: Hall effect. Hall voltageVHdivided by the currentIas a function of magnetic field for the 10 u. c. (black dots) and 15 u.c. (blue dots) LaTiO3/SrTiO3samples, measured at 100 mK. Red solid lines correspond to linear fits. (Inset)Tcas a function of doping for SrTiO3single crystals taken from reference27(black open circles). The two red dots correspond to LaTiO3/SrTiO3samples taking the thicknessd10 u.c.=12 nm,d15 u.c.=13.5 nm. Here, we have definedTcas the temperature at which the resistance reaches zero as this definition is more appropriate for comparison with the magnetic definition of theTcused in reference27. Errors bars represent the uncertainty in the comparison of the two definitions ofTc. Figure 4: Hall effect. Hall voltage V H divided by the current I as a function of magnetic field for the 10 u. c. (black dots) and 15 u.c. (blue dots) LaTiO 3 /SrTiO 3 samples, measured at 100 mK. Red solid lines correspond to linear fits. (Inset) T c as a function of doping for SrTiO 3 single crystals taken from reference [27] (black open circles). The two red dots correspond to LaTiO 3 /SrTiO 3 samples taking the thickness d 10 u.c. =12 nm, d 15 u.c. =13.5 nm. Here, we have defined T c as the temperature at which the resistance reaches zero as this definition is more appropriate for comparison with the magnetic definition of the T c used in reference [27] . Errors bars represent the uncertainty in the comparison of the two definitions of T c . Full size image It is known that LaTiO 3 itself can be oxygen [20] , [22] , [21] or Sr doped [23] , and thus becomes metallic. The key question is therefore: does superconductivity take place within a doped Mott insulator layer, namely oxygen- or Sr-doped LaTiO 3 , or within a 2-DEG formed at the LaTiO 3 /SrTiO 3 interface, which extends mostly within the band insulator SrTiO 3 (ref. 8 )? And conversely, do the electronic correlations, which are known to be strong in the former case and moderate in the latter one [16] , have a role in that context? The recent works on LaTiO 3 /SrTiO 3 superlattices [6] , [11] , [24] clearly indicate that under proper growth conditions, the interface is abrupt, with no sizable Sr diffusion for deposition temperatures below 1,000 °C [10] Optical spectroscopy confirms that the carrier properties in superlattices are different from the ones in La 1− x Sr x TiO 3 compounds [11] . Moreover, the low-temperature transport properties are different in conducting doped LaTiO 3 and doped SrTiO 3 . In both cases, electron–electron collisions dominate the scattering events according to the Fermi liquid picture. Figure 1 shows that, in an intermediate regime temperature, the temperature dependence of the resistance is well fitted by a quadratic law R ( T )= AT 2 + R 0 where the coefficient A depends on the Landau parameters, and therefore on the carrier density and the effective mass m* [25] . We obtained A =0.27Ω/□ K 2 for the 10 u.c. sample and A =0.11Ω/□ K 2 for the 15 u.c. sample. In Table 1 , we summarize the different values of A found in the literature for doped LaTiO 3 and doped SrTiO 3 thin films and crystals and compare them to the values extracted from our experiment. The largest values of A reported in doped LaTiO 3 are on the order of 1×10 −9 Ω cm / K 2 before the system becomes insulating at low temperature (∂ R /∂ T <0 for T <100 K), whereas it is two orders of magnitude higher for doped SrTiO 3 . From the comparison, we see that the LaTiO 3 /SrTiO 3 interface layer behave more like doped SrTiO 3 than doped LaTiO 3 . These observations are consistent with an electronic reconstruction of the LaTiO 3 /SrTiO 3 interface, leading to the formation of a few unit cells thick 2-DEG in the SrTiO 3 that projects mostly towards the SrTiO 3 substrate and makes it conducting layer [8] , [15] , [16] . As shown in Figure 4 inset, our data are consistent with the dependence of T c with the carrier density of doped SrTiO 3 reported in the literature [27] . Table 1 Comparison of A parameters (given in Ω cm / K 2 ) measured in the 10 u.c. and 15 u.c. LaTiO 3 /SrTiO 3 samples (taking the thickness d 10u.c. =12 nm, d 15u.c. =13.5 nm), with data obtained from literature on thin films and crystals for similar doping. Full size table In summary, we have measured the electronic transport properties of LaTiO 3 /SrTiO 3 heterostructures. The samples show a metallic behaviour and a superconducting transition is observed at low temperature. Our analysis shows that a 2-DEG is formed at the interface which is located mostly on the SrTiO 3 substrate, in agreement with the electronic reconstruction scenario [8] . This discovery opens the possibility to study the interplay between superconductivity and different electronic orders predicted to take place with ultra-thin LaTiO 3 films on SrTiO 3 . According to our results in terms of carrier density, mobility and gas thickness, it should be possible to modulate significantly the behaviour of the 2-DEG by adjusting the number of charge carriers with an electrostatic gate. Growth of LaTiO 3 /SrTiO 3 heterostructures We have grown epitaxial layers of LaTiO 3 using excimer laser-based PLD on commercially available (Crystal) single-crystal substrates of SrTiO 3 cut along (100) and (110) crystallographic directions. Although the (100) subtrates were given a buffered HF treatment to expose TiO 2 -terminated surface, the (110) plane has Sr, Ti and oxygen ions on one plane and hence HF treatment is irrelevant in this case. The substrates were glued to the heater block of the PLD system and heated in oxygen pressure of 200 mtorr in the temperature range of 850–950 °C for 1 h to realize surface reconstruction. This process has been used routinely to grow epitaxial films and heterostructures of YBa 2 Cu 3 O 6 + x and hole-doped manganites. The source of LaTiO 3 is a stoichiometric sintered target of 22 mm in diameter that was ablated in oxygen partial pressure of 1×10 −4 torr with energy fluence of ~1 J cm −2 per pulse at a repetition rate of 3 Hz to realize a gowth rate of 0.12 Å s −1 . X-ray characterizations The X-ray diffraction pattern of LaTiO 3 films deposited on (100) substrate is shown in Supplementary Figure S1 . After subtracting the contribution of the substrate, the lattice parameter of the film is found to be 3.956 Å (inset), in good agreement with previous studies [28] and close to the one reported in bulk LaTiO 3 (3.928 Å) [29] . The X-ray diffraction pattern ( θ −2 θ scan) around 32° of LaTiO 3 films deposited on SrTiO 3 (110) is shown in panel a of Supplementary Figure S2 . The (110) peak of the film is observed at 2 θ =32.193°, close to the (110) peak of the substrate, which corresponds to a LaTiO 3 lattice parameter of 3.928 Å. As shown in panel b of Supplementary Figure S2 , the typical width of the rocking curve of the (110) peak is about 0.1° indicating a very good out-of-plane orientation of the layers. How to cite this article: Biscaras, J. et al . Two-dimensional superconductivity at a Mott insulator/band insulator interface LaTiO 3 /SrTiO 3 . Nat. Commun. 1:89 doi: 10.1038/ncomms1084 (2010).